egoccupancy as an effective descriptor for the catalytic activity of perovskite oxide-based peroxidase mimics A peroxidase catalyzes the oxidation of a substrate with a peroxide. The search for peroxidase-like and other enzyme-like nanomaterials (called nanozymes) mainly relies on trial-and-error strategies, due to the lack of predictive descriptors. To fill this gap, here we investigate the occupancy of e g orbitals as a possible descriptor for the peroxidase-like activity of transition metal oxide (including perovskite oxide) nanozymes. Both experimental measurements and density functional theory calculations reveal a volcano relationship between the e g occupancy and nanozymes’ activity, with the highest peroxidase-like activities corresponding to e g occupancies of ~1.2. LaNiO 3- δ , optimized based on the e g occupancy, exhibits an activity one to two orders of magnitude higher than that of other representative peroxidase-like nanozymes. This study shows that the e g occupancy is a predictive descriptor to guide the design of peroxidase-like nanozymes; in addition, it provides detailed insight into the catalytic mechanism of peroxidase-like nanozymes. Artificial enzymes aim to imitate the unique catalytic activities of natural enzymes using alternative materials. Recently, functional nanomaterials with enzyme-like catalytic activities, called nanozymes, have emerged as promising alternatives that could overcome the low stability and high cost of natural enzymes [1] , [2] , [3] , [4] , [5] , [6] , [7] , [8] , [9] , [10] , [11] , [12] , [13] . Intriguingly, nanozymes are superior to molecular and polymeric enzyme mimics in several ways, such as their tunable catalytic activities, large surface areas for bioconjugation, and multiple functionalities in addition to catalysis [14] . Among different nanozymes, enormous efforts have been devoted to developing nanomaterials with peroxidase-like activity (i.e., \({\mathrm{AH}}_{\mathrm{2}} + {\mathrm{H}}_{\mathrm{2}}{\mathrm{O}}_{\mathrm{2}}\frac{{{\mathrm{Peroxidase - like}}}}{{{\mathrm{nanozyme}}}}{\mathrm{A}} + {\mathrm{2H}}_{\mathrm{2}}{\mathrm{O}}\) ) because of their broad applications, which range from biomedical diagnosis and bioimaging to antibacterial agents and antibiofouling coatings for medical devices [1] , [2] , [4] , [7] , [10] , [14] , [15] , [16] , [17] , [18] . Many nanomaterials, including systems based on various transition metal oxides (TMOs), have been explored as possible peroxidase mimics [14] . For example, Yan and colleagues [1] , [2] , [19] discovered the unexpected peroxidase-like activity of iron oxide nanoparticles, which were then applied to Ebola detection and tumor immunostaining. We have recently developed Ni oxide-based peroxidase mimics for glucose detection in serum [20] . However, these peroxidase-like nanozymes are generally developed using trial-and-error strategies [14] . The prevalence of empirical approaches is due to the lack of predictive descriptors—structural characteristics of the nanomaterials that can be used as proxies for their peroxidase-like activities. This lack of predictive descriptors significantly hampers the identification of more active nanozymes. Recently, several studies have demonstrated that for electrocatalysis and photocatalysis, the d -band center of metals, O 2 p -band center of TMOs, and e g occupancy of TMOs serve as suitable activity descriptors to design efficient electro- and photo-catalysts, respectively [21] , [22] , [23] , [24] , [25] , [26] , [27] , [28] , [29] , [30] , [31] , [32] , [33] , [34] , [35] , [36] , [37] , [38] . However, the activity descriptors of the enzyme-mimicking nanocatalysts (e.g., peroxidase-like nanozymes) remain largely unknown [39] . In this study, we aim to identify a predictive descriptor for TMO-based peroxidase mimics. We reason that the e g occupancy (i.e., the d -electron population of the e g (σ*) antibonding orbitals associated with the transition metal sites) may control the peroxidase-like activity of perovskite TMOs because of the central role of oxygen species in these biomimetic catalytic reactions. We choose ABO 3 -type perovskite TMOs with BO 6 octahedral subunits (where A is a rare earth or alkaline-earth metal and B is a transition metal) as a model system due not only to their low cost and ease of preparation, but, more importantly, also to their diverse and controllable structural and catalytic properties (Fig. 1a ) [24] , which may facilitate the tuning of the e g occupancy by adjusting the ABO 3 composition. We show that the peroxidase-like activity of ABO 3 -type perovskite TMOs is primarily governed by their e g occupancy. In particular, we identify a volcano relationship between the e g occupancy and the specific catalytic activity of perovskite TMO-based peroxidase mimics: namely, perovskite TMOs with an e g occupancy of ~1.2 and 0 (or 2) exhibit the highest and the lowest peroxidase-like activity, respectively. These conclusions are further rationalized by density functional theory (DFT) calculations. The identified descriptor successfully predicts the peroxidase-like activity of binary TMOs with octahedral coordination geometries. Fig. 1 Fe-based perovskite TMOs as peroxidase mimics. a Schematic of ABO 3 perovskite structure. A (rare earth or alkaline-earth metal), B (transition metal), and O are shown in gray, blue, and yellow, respectively. b 3 d electron occupancy of t 2g ( π *) and e g ( σ *) antibonding orbitals associated with the transition metal, for LaFeO 3 , La 0.5 Sr 0.5 FeO 3- δ , and SrFeO 3- δ . c TEM image of LaFeO 3 . Scale bar: 200 nm. d PXRD patterns of LaFeO 3 , La 0.5 Sr 0.5 FeO 3- δ , and SrFeO 3- δ (the red lines at the bottom mark the reference pattern of LaFeO 3 from the JCPDS database, card number 75-0541). e Typical absorption spectra of 0.8 mM TMB after catalytic oxidation with 50 mM H 2 O 2 in pH 4.5 acetate buffer at 40 °C, in the presence of 10 μg mL −1 of LaFeO 3 , La 0.5 Sr 0.5 FeO 3- δ , and SrFeO 3- δ nanozymes. f Time evolution of absorbance at 652 nm (A 652 ) for monitoring the catalytic oxidation of 1 mM TMB with 100 mM H 2 O 2 in the presence of 10 μg mL −1 of LaFeO 3 , La 0.5 Sr 0.5 FeO 3- δ , and SrFeO 3- δ nanozymes. g Specific peroxidase-like activities of LaFeO 3 , La 0.5 Sr 0.5 FeO 3- δ , and SrFeO 3- δ . h Specific peroxidase-like activity of the Fe-based perovskite TMOs as a function of e g occupancy. Source data are provided as a Source Data file Full size image Identification of nanozyme activity descriptor The perovskite samples were prepared by a sol-gel method followed by annealing at the desired temperatures. The as-prepared perovskites were fully characterized by scanning electron microscope (SEM), transmission electron microscope (TEM), powder X-ray diffraction (PXRD), inductively coupled plasma-optical emission spectroscopy (ICP-OES) and Brunauer–Emmett–Teller (BET) surface area measurements (see Supplementary Figs 1 – 13 and Supplementary Tables 1 – 2 for details). The amount of oxygen vacancies in the perovskites was quantified by iodometric titrations (Supplementary Table 3 ). To identify a suitable descriptor for the peroxidase-like activity of perovskite TMOs, we initially examined La 1- x Sr x FeO 3- δ compositions ( x = 0–1), because the e g occupancy of Fe in this series of perovskites could be gradually tuned by substituting La 3+ with Sr 2+ cation (Fig. 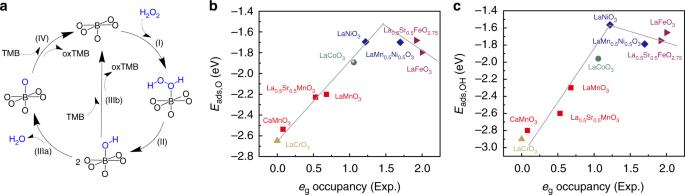Fig. 3 Computational analysis of the peroxidase-mimicking activity of ABO3perovskite TMOs.aProposed sub-processes responsible for the oxidation of TMB tooxTMB with the (001) facet of ABO3as peroxidase mimics.b,cAdsorption energies of O (Eads,O) and OH (Eads,OH) plotted as a function ofegoccupancy, whereEadsandegoccupancy were obtained by calculations and experiments, respectively. Source data are provided as a Source Data file 1b and Supplementary Table 4 ). Such a substitution would shift the oxidation state of Fe from + 3 in LaFeO 3 to + 3.31 in SrFeO 3- δ , resulting in the corresponding change of the e g occupancy of Fe from 2 to 1.69 (note: as there are no fractional electrons occupying these orbitals, the e g occupancies presented in the current study are averages between integer occupations). 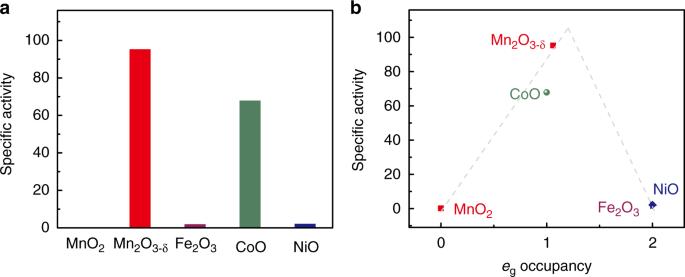Fig. 4 Binary TMOs as peroxidase mimics.aSpecific peroxidase-like activities of MnO2, CoO, Mn2O3-δ, NiO, and Fe2O3.bSpecific peroxidase-like activities of the binary metal oxides as a function ofegoccupancy. The two lines are shown for eye-guiding only. Source data are provided as a Source Data file A representative TEM image of LaFeO 3 (Fig. 1c ) reveals the typical irregular morphology of perovskites with nanoscale features. The formation of phase-pure La 1- x Sr x FeO 3- δ ( x = 0, 0.5, and 1) perovskite structures was confirmed by matching their PXRD data to the standard pattern of LaFeO 3 (JCPDS card number 75-0541) (Fig. 1d ). The peroxidase-like activity of the perovskite-based nanozymes was assessed by using absorption spectroscopy to monitor the catalytic oxidation of 3,3′,5,5′-tetramethylbenzidine (TMB, a typical peroxidase substrate) with H 2 O 2 in the presence of the nanozymes. The oxidation of TMB generates an oxidized product ( ox TMB) with a characteristic absorption peak at 652 nm. The intensity of this absorption peak (A 652 ) increased with increasing Sr content and the highest absorption was obtained for SrFeO 3- δ (Fig. 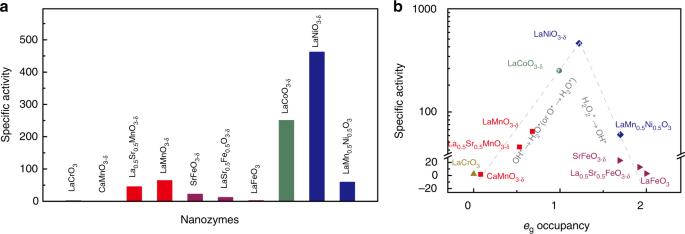1e ). The time evolution of the A 652 value (Fig. 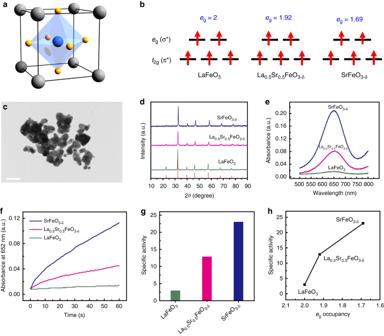Fig. 2 Evaluation ofegoccupancy as an effective descriptor for catalytic activity of perovskite TMO-based peroxidase mimics.aSpecific peroxidase-like activities of perovskite TMOs.bSpecific peroxidase-like activities of perovskite TMOs plotted as a function ofegoccupancy, in which equations shown in gray are the rate-limiting reaction steps (note: the rate-limiting steps of the catalytic reaction would be discussed in DFT calculations section). The two lines are shown for eye-guiding only. Source data are provided as a Source Data file 1f ) shows that SrFeO 3- δ also exhibited the fastest reaction kinetics, demonstrating that the Sr substitution effectively enhanced the peroxidase-like activity of La 1- x Sr x FeO 3- δ . The mass-based peroxidase-like activities of nanozymes were measured by steady-state kinetics assays (see Methods section). Fig. 1 Fe-based perovskite TMOs as peroxidase mimics.aSchematic of ABO3perovskite structure. A (rare earth or alkaline-earth metal), B (transition metal), and O are shown in gray, blue, and yellow, respectively.b3delectron occupancy oft2g(π*) andeg(σ*) antibonding orbitals associated with the transition metal, for LaFeO3, La0.5Sr0.5FeO3-δ, and SrFeO3-δ.cTEM image of LaFeO3. Scale bar: 200 nm.dPXRD patterns of LaFeO3, La0.5Sr0.5FeO3-δ, and SrFeO3-δ(the red lines at the bottom mark the reference pattern of LaFeO3from the JCPDS database, card number 75-0541).eTypical absorption spectra of 0.8 mM TMB after catalytic oxidation with 50 mM H2O2in pH 4.5 acetate buffer at 40 °C, in the presence of 10 μg mL−1of LaFeO3, La0.5Sr0.5FeO3-δ, and SrFeO3-δnanozymes.fTime evolution of absorbance at 652 nm (A652) for monitoring the catalytic oxidation of 1 mM TMB with 100 mM H2O2in the presence of 10 μg mL−1of LaFeO3, La0.5Sr0.5FeO3-δ, and SrFeO3-δnanozymes.gSpecific peroxidase-like activities of LaFeO3, La0.5Sr0.5FeO3-δ, and SrFeO3-δ.hSpecific peroxidase-like activity of the Fe-based perovskite TMOs as a function ofegoccupancy. Source data are provided as a Source Data file To separate the effect of surface area from the intrinsic peroxidase-like activity of perovskites (including the Fe-based perovskites discussed in this section), their specific activity (i.e., the mass activity normalized to the surface area) was also calculated, based on the BET surface areas obtained by nitrogen desorption measurements (Supplementary Figs 3 and 6 , and Supplementary Table 1 ). As shown in Fig. 1g , the specific activity of SrFeO 3- δ was 7.76 and 1.79 times higher than that of LaFeO 3 and La 0.5 Sr 0.5 FeO 3- δ , respectively. The dependence of the specific activity on the Sr content of La 1- x Sr x FeO 3- δ and the e g occupancy of Fe is plotted in Fig. 1h . A substantial improvement in the peroxidase-like activity of La 1- x Sr x FeO 3- δ was observed as the Sr content increased from 0 to 1 and the e g occupancy of Fe decreased from 2 to 1.69. To study the effect of e g occupancy lower than 1 on the peroxidase-like activity of perovskites, we investigated three Mn-based perovskites with the e g occupancy of Mn varying from 0.68 to ~0.08 (i.e., e g = 0.68, 0.53, and 0.08 for LaMnO 3- δ , La 0.5 Sr 0.5 MnO 3- δ , and CaMnO 3- δ , respectively). The SEM and TEM images shown in Supplementary Figs 4 and 5 , and the PXRD patterns in Supplementary Fig. 7a demonstrate the successful synthesis of the Mn-based perovskites. As shown in Supplementary Fig. 7c , the specific activity of LaMnO 3- δ was 1.42 and 43.29 times higher than that of La 0.5 Sr 0.5 MnO 3- δ and CaMnO 3- δ , respectively. Supplementary Fig. 7e shows the effect of the e g occupancy on the specific peroxidase-like activity of the Mn-based perovskites. Different from the trend observed for the Fe-based perovskites (i.e., the peroxidase-like activity increased as the e g occupancy decreased), the catalytic activity of the Mn-based perovskites decreased as the e g occupancy further decreased from 0.68 to ~0.08. Taken together, the above results show a strong but non-monotonic correlation between e g occupancy and peroxidase-like activity of perovskites, suggesting the e g occupancy as a potential activity descriptor. Evaluation of e g occupancy as nanozyme activity descriptor To further evaluate the correlation between the e g occupancy and their peroxidase-like activity, overall ten perovskite TMOs covering e g occupancies of 0–2, six as described above and four others (i.e., LaCrO 3 , LaCoO 3- δ , LaNiO 3- δ , and LaMn 0.5 Ni 0.5 O 3 ) were investigated (Supplementary Figs 8 – 14 , Supplementary Table 6 , and Supplementary Notes 1–2 ). As shown in the summary in Fig. 2a , the perovskite TMOs exhibited significantly different specific peroxidase-like activities. Some of them (such as LaNiO 3- δ ) exhibited a high activity, whereas the activity of others (such as LaCrO 3 ) was negligible. This behavior can be understood by plotting the activities of the ten perovskite TMOs as a function of the corresponding e g occupancy associated with the B cations: a definitive volcano relationship is obtained (Fig. 2b ). The mass-based peroxidase-like activities (i.e., mass activities) of the perovskite TMOs also show a volcano dependence on the corresponding e g occupancies (Supplementary Fig. 15 ), confirming that the catalytic activity of the perovskite TMO-based peroxidase mimics is primarily governed by the e g occupancy of the B cations. In particular, perovskite TMOs with e g occupancy of ~1.2 exhibit the highest peroxidase-like activity (Fig. 2 ). Fig. 2 Evaluation of e g occupancy as an effective descriptor for catalytic activity of perovskite TMO-based peroxidase mimics. a Specific peroxidase-like activities of perovskite TMOs. b Specific peroxidase-like activities of perovskite TMOs plotted as a function of e g occupancy, in which equations shown in gray are the rate-limiting reaction steps (note: the rate-limiting steps of the catalytic reaction would be discussed in DFT calculations section). The two lines are shown for eye-guiding only. Source data are provided as a Source Data file Full size image Evaluation of other parameters as potential descriptors As several other potential descriptors (i.e., oxidation state of transition metal, 3 d electron number of B-site ions, O 2 p -band center, and B-O covalency) have been studied to predict the electrocatalytic and photocatalytic activities of perovskites, we also investigated the relationship between the peroxidase-like activity and these parameters. As shown in Supplementary Fig. 16 , although the oxidation state of B sites affects the peroxidase-like activity of perovskites, there is no apparent relationship between them. These results indicated that the oxidation state of B sites is not an effective descriptor and cannot provide guidance for the rational design of peroxidase-like nanozymes. We then studied the relationship between the peroxidase-like activity and the 3 d electron number of B-site ions. As shown in Supplementary Fig. 17 , an “M-shaped” relationship with the maximum peroxidase-like activities around d 4 and d 7 was obtained. Clearly, although the 3 d electron number is indicative, it is not a straightforward descriptor, as two maxima are associated with it. Several recent studies suggested that the O 2 p -band center could be a better activity descriptor than the e g occupancy to design catalysts for oxygen reduction reaction and oxygen evolution reaction [33] , [34] , [40] ; therefore, we also evaluated it as a potential descriptor for the peroxidase-like activity of perovskites (Supplementary Note 6 ). As shown in Supplementary Fig. 18 , the O 2 p -band center was not well correlated with the peroxidase-like activity of perovskites, suggesting that it is not an effective descriptor for the perovskite-based peroxidase mimics. Last, we studied the relationship between the peroxidase-like activity and B-O covalency. The B-O covalency was approximately quantified by the normalized O 1 s → B 3 d – O 2 p absorbance from O K-edge X-ray absorption spectra [21] . As shown in Supplementary Fig. 19 , there is no apparent relationship between the B-O covalency and the peroxidase-like activity of the six representative perovskites. Interestingly, for the perovskites with e g occupancy close to 1 (i.e., LaMnO 3- δ , LaCoO 3- δ , and LaNiO 3- δ ), their peroxidase-like activity increases with the increasing of covalency strength of B-O. These results suggested that the B-O covalency may act as a secondary descriptor for peroxidase-like activity when the e g occupancy of B-site is close to 1 (Supplementary Note 3 ). In short, in contrast to the e g occupancy, none of the four parameters discussed in this section showed a volcano relationship with the peroxidase-like activity of perovskites. These results further validated that the e g occupancy as an effective activity descriptor to predict the peroxidase-like activity of perovskites. DFT calculations To theoretically explain the effect of e g occupancy on the peroxidase-like activity, we performed DFT calculations for 11 ABO 3 perovskites (i.e., LaCrO 3 , CaMnO 3 , La 0.5 Sr 0.5 MnO 3 , LaMnO 3 , LaCoO 3 , LaNiO 3 , SrFeO 3 , LaMn 0.5 Ni 0.5 O 3 , La 0.5 Sr 0.5 FeO 2.75 , LaFeO 3 , and La 0.5 Sr 0.5 FeO 3 ) and proposed molecular mechanisms for the activities. The calculated geometric parameters and e g occupancy values for these bulk structures generally agreed with the experimental ones (Supplementary Table 9 and Supplementary Figs 20 – 22 ). We proposed that these perovskites mimicked peroxidases via mechanisms of Fig. 3a : (1) the adsorption (I) and dissociation (II) of H 2 O 2 molecules on ABO 3 surfaces to generate the OH adsorption species; (2) the conversion of these OH adsorption species to O adsorption species, which subsequently oxidize TMB substrates (IIIa and IV); (3) or alternatively, the direct oxidization of TMB by the OH adsorption species (IIIb). Perovskite ABO 3 (001) surfaces with the BO 2 termination were selected as the surfaces of reactions, because transition metal B in these surfaces are all five coordinated and each has one open coordination site. The five coordinated BO 2 termination is analogous to metals in metalloporphyrins, the active centers of many natural enzymes. The adsorption of H 2 O 2 on perovskite (001) surfaces has no energy barriers (Supplementary Fig. 23 ), suggesting step I does not determine the overall reaction rate. The variations of absorption energies ( E ads ) for O ( E ads,O ) and OH ( E ads,OH ) with respect to e g occupancy are shown in Fig. 3b, c , and that for H 2 O 2 ( \(E_{{\mathrm{ads}},\, {\mathrm{H}}_{2}{\mathrm{O}}_{2}}\) ) in Supplementary Fig. 24 . Volcano-like relationships were found for E ads,O and E ads,OH with e g occupancy (Fig. 3b and c and Supplementary Fig. 24 ). Further analysis shows that the five perovskites with e g occupancy < 1.2 (i.e., LaCrO 3 , CaMnO 3 , La 0.5 Sr 0.5 MnO 3 , LaMnO 3 , and LaCoO 3 ) have strong OH* and O* adsorption energies; the other five perovskites with e g occupancy > 1.2 (i.e., LaMn 0.5 Ni 0.5 O 3 , SrFeO 3 , La 0.5 Sr 0.5 FeO 2.5 , La 0.5 Sr 0.5 FeO 3 , and LaFeO 3 ) as well as LaNiO 3 have weak OH* and O* adsorption energies. Perovskites with e g occupancy of ~1.2 have the weakest O and OH adsorption, in which the transfer of these oxygen species to TMB substrates is the easiest, in agreement with their highest peroxidase-mimicking activities. However, LaFeO 3 with negligible peroxidase-like activity also possesses weak O and OH adsorption. Therefore, we reasoned that the oxidation of the substrate (i.e., IIIb and IV of Fig. 3a ) is not the only rate-determining step. Reportedly, when a kinetic profile goes through a maximum as a function of a given parameter, it means that there is a change of the rate-determining step governing the reaction mechanism [32] . To identify all the rate-determining steps and to validate the mechanisms of Fig. 3a , we further calculated the energies for species involved in the proposed reaction pathways (Supplementary Figs 23 – 25 ). Supplementary Fig. 25 plots the energies of species involved in the proposed reaction pathways. It reveals that for the five perovskites with e g occupancy < 1.2, which are all located on the left side of Fig. 2b ’s volcano-like plots, the rate-determining step should be the oxidation of the substrate (i.e., IIIb and IV of Fig. 3a ); for the other five with e g occupancy > 1.2, which are all located on the right side of the volcano-like plots, the rate-determining step should be the O–O bond splitting of the adsorbed H 2 O 2 * (II of Fig. 3a ); LaNiO 3 is the maximum point where the rate-determining step changes. Taking these results together, e g occupancy influences the peroxidase-mimicking activities of perovskites by altering the E ads of reaction intermediates and the rate-determining step governing the catalytic reactions. Perovskites with e g occupancy of ~1 possess optimal E ads and can facilitate these rate-determining steps efficiently, which further lead to the high peroxidase-like activity. Fig. 3 Computational analysis of the peroxidase-mimicking activity of ABO 3 perovskite TMOs. a Proposed sub-processes responsible for the oxidation of TMB to ox TMB with the (001) facet of ABO 3 as peroxidase mimics. b , c Adsorption energies of O ( E ads,O ) and OH ( E ads,OH ) plotted as a function of e g occupancy, where E ads and e g occupancy were obtained by calculations and experiments, respectively. Source data are provided as a Source Data file Full size image General applicability of the e g occupancy To test whether e g occupancy could also predict the activity of non-perovskites TMOs with the same metal-oxygen octahedral coordination geometry as the perovskites described above, we investigated the peroxidase-like activity of five binary metal oxide nanoparticles (Supplementary Figs 26 – 28 , Supplementary Table 7 , and Supplementary Note 4 ). First, to demonstrate the predictive power of the descriptor, CoO and Mn 2 O 3-δ nanoparticles with unit e g occupancy were tested, as their peroxidase-like activities are unknown. If the e g occupancy descriptor was also applicable to the binary metal oxides, these nanoparticles would be expected to exhibit high peroxidase-like activities. As shown in Supplementary Figs 29 , 30a and Fig. 4a , both nanoparticles exhibited excellent activities, in agreement with the prediction based on the e g occupancy descriptor. By contrast, the measured peroxidase-like activities of MnO 2 ( e g = 0), Fe 2 O 3 ( e g = 2), and NiO ( e g = 2) nanoparticles were nearly negligible (Supplementary Fig. 29 and Fig. 4a ), again in agreement with the prediction. These results clearly demonstrate that the peroxidase-like activity of binary metal oxides with octahedral coordination geometry is similarly associated with the e g occupancy, with a similar volcano dependence to that obtained for the perovskite TMO-based peroxidase mimics (Supplementary Fig. 30b and Fig. 4b ). Fig. 4 Binary TMOs as peroxidase mimics. a Specific peroxidase-like activities of MnO 2 , CoO, Mn 2 O 3-δ , NiO, and Fe 2 O 3 . b Specific peroxidase-like activities of the binary metal oxides as a function of e g occupancy. The two lines are shown for eye-guiding only. Source data are provided as a Source Data file Full size image Comparison with other peroxidase mimics Among the 16 TMOs studied in this work (Figs 2 , 4 and Supplementary Fig. 10 ), LaNiO 3- δ was identified as the most active peroxidase mimic, in terms of both specific and mass activities (Supplementary Note 5 ). Over the last decade, dozens of nanomaterials have been proposed as peroxidase mimics [41] . A comparison between the nanozymes developed in this work and those reported in the literature may be useful for searching for new nanozymes. However, a direct comparison between data produced by different studies is difficult, because the applied protocols or even the specific test conditions, such as temperature and H 2 O 2 concentration, could significantly influence the peroxidase-like activity of the nanomaterials. To allow for a reliable and rigorous comparison, we synthesized several peroxidase mimics reported in previous studies (Fig. 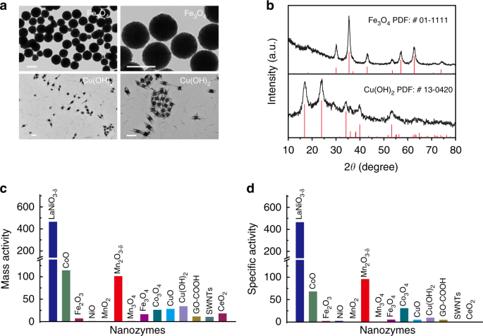Fig. 5 Comparison of peroxidase-like activity of LaNiO3-δand other nanozymes.aRepresentative TEM images of Fe3O4and Cu(OH)2at different magnifications. Scale bars: 500 nm.bPXRD patterns of Fe3O4and Cu(OH)2(the red lines mark the reference patterns of Fe3O4(JCPDS card number 01-1111) and Cu(OH)2(JCPDS card number 13-0420)).cMass-normalized peroxidase-like activities of LaNiO3-δand other nanozymes.dSpecific peroxidase-like activities of LaNiO3-δand other nanozymes. Source data are provided as a Source Data file 5 , Supplementary Methods, Supplementary Figs 26 – 28 , 31 – 32 , and Supplementary Table 5 ) and compared their peroxidase-like activities with that of LaNiO 3- δ under the same conditions. Fe 3 O 4 nanoparticles and Cu(OH) 2 supercages were chosen as representative peroxidase mimics for comparison: Fe 3 O 4 nanoparticles were the first reported peroxidase mimics, whereas Cu(OH) 2 supercages are the state-of-the-art representatives of these systems, with K cat (catalytic constant) values comparable to those of natural peroxidase [1] , [42] . Fig. 5a,b confirm the successful preparation of Fe 3 O 4 nanoparticles and Cu(OH) 2 supercages. The time evolution of the A 652 parameter (Supplementary Fig. 33 and Fig. 5c ) shows that the mass activity of LaNiO 3- δ is 28.9 and 13.6 times higher than that of the Fe 3 O 4 nanoparticles and Cu(OH) 2 supercages, respectively. Moreover, Fig. 5d shows that the specific activity of LaNiO 3- δ was 91.4 and 49.0 times higher than that of the Fe 3 O 4 nanoparticles and Cu(OH) 2 supercages, respectively, because of the smaller surface area of the LaNiO 3- δ nanoparticles prepared by the sol-gel method. Other representative nanozymes (such as CeO 2 , CuO, single-walled carbon nanotubes, and graphene oxide (GO-COOH)) were also investigated. The results in Fig. 5c,d confirm the superior performance of LaNiO 3- δ , in terms of both specific and mass activity, further demonstrating the power of the e g occupancy descriptor for identifying nanozymes of particularly high activity. Fig. 5 Comparison of peroxidase-like activity of LaNiO 3- δ and other nanozymes. a Representative TEM images of Fe 3 O 4 and Cu(OH) 2 at different magnifications. Scale bars: 500 nm. b PXRD patterns of Fe 3 O 4 and Cu(OH) 2 (the red lines mark the reference patterns of Fe 3 O 4 (JCPDS card number 01-1111) and Cu(OH) 2 (JCPDS card number 13-0420)). c Mass-normalized peroxidase-like activities of LaNiO 3- δ and other nanozymes. d Specific peroxidase-like activities of LaNiO 3- δ and other nanozymes. Source data are provided as a Source Data file Full size image Using experimental measurements and DFT calculations, we have identified the e g occupancy as a predictive and effective descriptor for the peroxidase-like activity of TMO (including perovskite TMO) nanomaterials. The catalytic activity of peroxidase-like nanozymes with metal-oxygen octahedral coordination geometry shows a volcano dependence on the e g occupancy. Namely, nanozymes with e g occupancy of ~1.2 had the highest catalytic activity, whereas e g occupancies of 0 or 2 corresponded to negligible activities. The systematic comparison of more than 20 representative peroxidase-like nanozymes revealed that LaNiO 3- δ had the highest catalytic activity. Besides supporting an approach to the design of highly active peroxidase mimics based on the e g occupancy, the present study also provided deep insight into the catalytic mechanism of the peroxidase-like activity of the nanozymes. Taking into account the adaptable structures and catalytic activities of TMO-based nanozymes, the current study has prompted us to further explore the application of the e g occupancy descriptor to predict the enzyme-like activities of other metal oxides. Synthesis of perovskite TMOs The perovskite TMOs were synthesized via a sol-gel method [43] . Briefly, the respective metal nitrate salts in appropriate stoichiometric ratios (3 mmol in total) and citric acid (12 mmol) were dissolved in 100 mL of H 2 O, followed by the addition of 1.5 mL of ethylene glycol. The resulting transparent solutions were treated at 90 °C under stirring to condense them into gel, which were then decomposed at 180 °C for 5 h to form the solid precursors. The latter were decomposed at 400 °C for 2 h to remove the organic components and obtain foam precursors, which were further annealed at 700 °C (850 °C in the case of CaMnO 3- δ ) for 5 h with a ramp rate of 5 °C min −1 , to obtain the final perovskite TMOs. Structure characterization PXRD data were collected at room temperature using a Rigaku Ultima diffractometer using Cu Kα radiation. The diffractometer was operated at 40 kV and 40 mA, with a scan rate of 5° min −1 and a step size of 0.02°. TEM images were recorded on a JEOL JEM-2100 or FEI Tecnai F20 microscope at an acceleration voltage of 200 kV. SEM measurements were performed on a Hitachi S-4800 microscope operated at 5 kV. UV-visible absorption spectra were collected using a spectrophotometer (TU-1900, Beijing Purkinje General Instrument Co. Ltd, China). Nitrogen adsorption–desorption isotherms were measured at 77 K using a Quantachrome Autosorb-IQ-2C-TCD-VP analyzer and were used to calculate the surface areas of the nanozymes with the BET method. The temperature-dependent magnetization was measured on a MPMS SQUID magnetometer (MPMS-3, Quantum Design) with a magnetic field of H = 1 kOe under field-cooling procedures. O K-edge X-ray absorption spectroscopy (XAS) measurements were performed at the beamline BL12B-a (CMD) in Hefei Synchrotron Radiation Facility, National Synchrotron Radiation Laboratory. Peroxidase-like activity measurements Steady-state kinetics assays were conducted at 37 °C in 1.0 mL cuvettes with a path length of 0.2 cm. A 0.2 M NaOAc buffer solution (pH 4.5) was used as the reaction buffer and 10 μg mL −1 of nanozymes were used for their kinetics assays. The kinetics data were obtained by varying the concentration of H 2 O 2 while keeping the TMB’s concentration constant (Supplementary Table 8 ). The kinetics constants (i.e., v max and K m ) were calculated by fitting the reaction velocity values and the substrate concentrations to the Michaelis–Menten equation as follows: 
    v = v_max× [S]/K_m + [S]
 (1) where v is the initial reaction velocity and v max is maximal reaction velocity. v max is obtained under saturating substrate conditions. [ S ] is the substrate concentration. K m , the Michaelis constant, equals to the concentration of substrate when the initial reaction velocity reaches half of its maximal reaction rate. As for TMOs with negligible activity (i.e., LaCrO 3 , LaFeO 3 , CaMnO 3- δ , NiO, MnO 2 , and Mn 3 O 4 ), we assumed the initial reaction velocity in the presence of 10 μg mL −1 of nanozymes, 1 mM TMB, and 100 mM H 2 O 2 as the v max , because the kinetics measurements for them were difficult and not reliable. The mass activities of the nanozymes were defined as follows: 
    Mass activity = v_max
 (2) The specific activities of the nanozymes were calculated from Eqs ( 3 ) and ( 4 ): 
    Specific activity = Mass activity/Normalized BET area
 (3) 
    Normalized BET area = BET area of nanozyme/BET area of LaNiO_3 - δ
 (4) DFT calculations The bulk structure of each defect-free perovskite was modeled using the A 8 B 8 O 24 unit cell, which was sufficiently large to consider all possible G-type antiferromagnetic (G-AFM), A-type antiferromagnetic (A-AFM), and paramagnetic (PM) magnetic orderings previously reported for perovskites (Supplementary Fig. 20 ). Geometrically relaxed ground-state bulk structures were then used to build the (001) slabs, each of which contained six layers: three AO and three BO 2 (Supplementary Fig. 21 ). For geometry optimizations of bulks, their space group symmetries (Supplementary Table 9 ) were used to constrain the geometries. For geometry optimizations using slab models, atoms in the bottom two layers (i.e., one AO and one BO 2 layer) were frozen and those in the above layers were allowed to move; lattice parameters were frozen for calculations with slab models. The generalized gradient approximation with the Perdew–Burke–Ernzerhof functional [44] was used for all geometry optimizations and energy calculations, in a planewave basis set with an energy cut-off of 500 eV and Gaussian smearing of 0.05 eV. The Hubbard U correction, where U is defined as U eff , was applied for B metals of perovskites to treat the strong on-site Coulomb interaction of their localized d electrons (Supplementary Table 10 ) [45] , [46] , [47] . For calculations of bulks and slabs, the (3 × 3 × 3) and (3 × 3 × 1) Monkhorst−Pack [48] meshes were used for the k -point samplings, respectively. The convergence thresholds for the electronic structure and forces were set to be 10 −5 eV and 0.02 eV Å −1 , respectively. All calculations were performed using the VASP code [49] . More details of the computations can be found in Supplementary Note 6 .